Solar wind entry into the high-latitude terrestrial magnetosphere during geomagnetically quiet times An understanding of the transport of solar wind plasma into and throughout the terrestrial magnetosphere is crucial to space science and space weather. For non-active periods, there is little agreement on where and how plasma entry into the magnetosphere might occur. Moreover, behaviour in the high-latitude region behind the magnetospheric cusps, for example, the lobes, is poorly understood, partly because of lack of coverage by previous space missions. Here, using Cluster multi-spacecraft data, we report an unexpected discovery of regions of solar wind entry into the Earth’s high-latitude magnetosphere tailward of the cusps. From statistical observational facts and simulation analysis we suggest that these regions are most likely produced by magnetic reconnection at the high-latitude magnetopause, although other processes, such as impulsive penetration, may not be ruled out entirely. We find that the degree of entry can be significant for solar wind transport into the magnetosphere during such quiet times. The Earth is one of the six solar system planets that have global magnetic fields [1] , which are sufficient to block and deflect most solar wind charged particles from the Sun’s atmosphere, and prevent them from directly interacting with the atmosphere of the planet [2] , [3] . This shielding is thought to be one of the most important factors protecting life on the ground and spacecraft in geospace from being damaged [4] , [5] . A small portion of these charged particles penetrates into the terrestrial magnetosphere, the shielded region of geospace [6] , [7] , [8] , [9] , which enhances the magnetospheric populations in different regions through various processes dependant on prevailing conditions. Such particles participate in active magnetospheric, ionospheric and upper atmospheric processes, such as storms, substorms, aurorae and other space weather effects, which can be hazardous to satellites, communication networks, power facilities and navigation systems and can even threaten astronaut health [4] , [5] . An understanding of the transport of solar wind plasma throughout the terrestrial magnetosphere is, therefore, one of the most important issues in space science and space weather. The majority of these penetrating solar wind plasma are generally thought to enter through the low-latitude region, via the process of magnetic reconnection (MR) [10] , [11] , during active times when the interplanetary magnetic field (IMF) has a southward component. Although previous studies have demonstrated that enhanced amounts of plasma enter to form a relatively thick, low-latitude boundary layer [2] , [12] , [13] and a denser plasma sheet [13] , [14] when the IMF is northward even during quiet times, the dominant mechanism of solar wind entry into the magnetosphere (and entry location on the magnetopause) under these conditions is less clear and still controversial. It is still not very clearly understood whether the entering plasma is a result of the high-latitude MR [12] , [15] , [16] , [17] , [18] , [19] , [20] , [21] , [22] , impulsive penetration [23] , [24] , or from the low latitudes through instabilities [25] , [26] or gradient drift [27] . Moreover, properties in the high-latitude region behind the mid-altitude magnetospheric cusps are poorly understood, partly as a result of lack of coverage by investigative space missions. Previous observations have shown that the magnetospheric lobe [6] , [7] , which occupies the majority of the magnetotail volume in the high latitudes, typically forms a reservoir of magnetic energy [28] , consisting of tenuous, low energy ions of internal, ionospheric origin [7] , [29] . Although observations [30] and numerical simulations [20] , [21] , [22] have inferred that plasmas from outer regions, for example, compressed solar wind in the magnetosheath, may enter the high-latitude lobe regions, direct observations of these plasmas inside are rare, partly because high-latitude lobes tailward of the mid-altitude cusps have seldom been explored in situ , restricting our ability to gain an understanding of this region. The four-satellite Cluster mission, however, uniquely has both sufficient polar orbital coverage ( Fig. 1 ) in this region and has taken an unprecedented set of coordinated multi-point measurements. 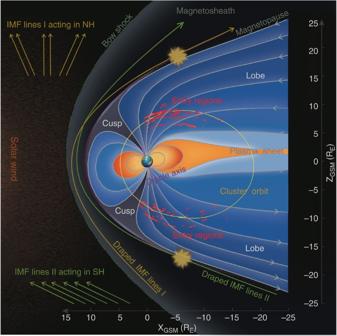Figure 1: Solar wind entry regions in the high-latitude terrestrial magnetosphere as detected by Cluster. Entry regions are indicated here as red markers. The C1 orbits and magnetospheric field lines are projected into the Geocentric Solar Magnetospheric (GSM) coordinate system XZ plane to indicate locations. The magnetospheric field lines are plotted according to the T89 model8, and the magnetopause and bow shock are based on models by Sibecket al.9with a 2 nPa solar wind dynamic pressure. Background colours illustrate different regions of the magnetosphere and the solar wind. The dipole orientation (tilting towards the Sun) corresponds to 12:00UT on 3rd September 2002 and one complete orbit of Cluster for that day are plotted with a yellow line. Here we show a possible process of the plasma entry. When the IMF is northward, MR between the IMF and magnetic field in the magnetosphere may occur at the high-latitude magnetopause. As the dipole axis is tilted towards the Sun, IMF field lines (orange) with any Bx sign can interact with the magnetospheric field lines in the northern hemisphere (NH), whereas only those IMFs with positive Bx values (green) are more likely to interact with the magnetospheric field lines in the southern hemisphere (SH). This leads to different IMF behaviour for the events in the NH and SH, as shown inFig. 4. Figure 1: Solar wind entry regions in the high-latitude terrestrial magnetosphere as detected by Cluster. Entry regions are indicated here as red markers. The C1 orbits and magnetospheric field lines are projected into the Geocentric Solar Magnetospheric (GSM) coordinate system XZ plane to indicate locations. The magnetospheric field lines are plotted according to the T89 model [8] , and the magnetopause and bow shock are based on models by Sibeck et al. [9] with a 2 nPa solar wind dynamic pressure. Background colours illustrate different regions of the magnetosphere and the solar wind. The dipole orientation (tilting towards the Sun) corresponds to 12:00UT on 3rd September 2002 and one complete orbit of Cluster for that day are plotted with a yellow line. Here we show a possible process of the plasma entry. When the IMF is northward, MR between the IMF and magnetic field in the magnetosphere may occur at the high-latitude magnetopause. As the dipole axis is tilted towards the Sun, IMF field lines (orange) with any Bx sign can interact with the magnetospheric field lines in the northern hemisphere (NH), whereas only those IMFs with positive Bx values (green) are more likely to interact with the magnetospheric field lines in the southern hemisphere (SH). This leads to different IMF behaviour for the events in the NH and SH, as shown in Fig. 4 . Full size image Using this data set, we report observations of several new solar wind plasma entry regions discovered in the high latitudes of the Earth’s magnetosphere, that is, the lobes tailward of the cusp region, during quiet times, as indicated in Fig. 1 . From several observational facts, as well as data analysis of global magnetohydrodynamics (MHD) simulation, we discuss several entry mechanisms and suggest a most possible one. As we explain below, the occurrence of these regions suggests that they are responsible for the majority of the plasma transport into the lobe region under these conditions. Solar wind origin plasmas in the high-latitude lobe We have used data taken between August and October each year from 2002–2004, when the Cluster spacecraft travelled from the dayside, through the mid-altitude cusp and high-latitude lobe into the plasma sheet (and thence through the southern hemisphere on its inbound leg), as summarized in Fig. 1 . Data from the Flux Gate Magnetometer [31] , Cluster Ion Spectrometry Experiment [32] and Plasma Electron and Current Experiment [33] instruments onboard Cluster have been used for this study. The time-shifted 1 min OMNI data at the earth’s bow shock is used to get the solar wind parameters and the IMF. 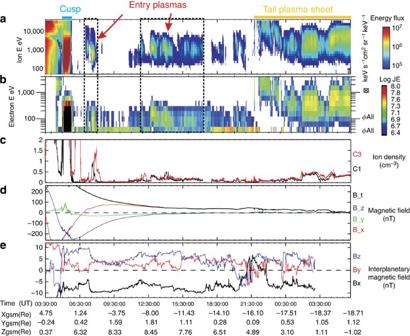Figure 2: One example for the entry plasmas observed at the high-latitude magnetosphere on 8 September 2002. (a) The hot ion energy spectrogram; (b) the electron energy spectrogram; (c) the hot ion density for C1 and C3; (d) the magnetic field in the GSM coordinate system, and (e) the solar wind magnetic field in GSM. The blue bar marks the duration for the cusp crossing, whereas the orange bar indicates the magnetotail plasma sheet. The high-latitude magnetosphere (where the lobe region is located), which is traditionally thought to have cold and tenuous plasmas with few entering solar wind plasmas, was observed between these two regions. The intervals of entry plasmas are indicated within this region and correspond to times when the solar wind magnetic field (d) is directed northward. More information can be found inSupplementary Fig. S1. Lowest threshold values of the energy flux are set to plot (a) and (b). Figure 2 shows an example. Within the high-latitude magnetosphere, there are certain locations with plasma populations that differ markedly from those of the background lobe population. The proton pitch angle distribution ( Supplementary Fig. S1b ) measured by Cluster is nearly isotropic for these locations and most of the protons have energies above several hundred electronvolts ( Fig. 2a ). Therefore, the character of these ion distributions is similar to those in the magnetosheath or cusp (regions filled with compressed solar wind plasma). There is also a decreased ratio of oxygen ion to proton number density ( Supplementary Fig. S1f ) within these events. As upflowing ions from the ionosphere normally consist of a large oxygen ion component [7] , [34] , this provides further evidence that the dominant portion of these ions (protons) is derived from the magnetosheath and not from the ionosphere. The data suggests, therefore, that these populations have entered at the high-latitude magnetopause during northward IMF ( Fig. 2e ). For this pass, the three other Cluster spacecraft have also observed this region with electron data [33] ( Fig. 2b , and Supplementary Fig. S1c,d,g ). In our previous studies [35] , [36] , we have reviewed a method on how to empirically distinguish the spatial ‘pass through’ effects from temporal ‘enter/retreat’ ones based on the temporal sequences of the four spacecraft. In summary, if we find ‘interlaced’ profiles of parameters observed by different spacecraft, it should be interpreted as a spatial ‘pass through’ structure. Then from Fig. 2c (and Supplementary Fig. S1g ), we have found that the time intervals containing the enhanced plasma represent a spatial zone moving towards lower latitudes. Figure 2: One example for the entry plasmas observed at the high-latitude magnetosphere on 8 September 2002. ( a ) The hot ion energy spectrogram; ( b ) the electron energy spectrogram; ( c ) the hot ion density for C1 and C3; ( d ) the magnetic field in the GSM coordinate system, and ( e ) the solar wind magnetic field in GSM. The blue bar marks the duration for the cusp crossing, whereas the orange bar indicates the magnetotail plasma sheet. The high-latitude magnetosphere (where the lobe region is located), which is traditionally thought to have cold and tenuous plasmas with few entering solar wind plasmas, was observed between these two regions. The intervals of entry plasmas are indicated within this region and correspond to times when the solar wind magnetic field ( d ) is directed northward. More information can be found in Supplementary Fig. S1 . Lowest threshold values of the energy flux are set to plot ( a ) and ( b ). Full size image Statistical survey of the entry regions To confirm the result of the case study, the occurrence of these entry regions is determined statistically by initially selecting those time periods when the Cluster satellites were in the high-latitude lobe. The boundary from the lobe to the plasma sheet was defined by the plasma beta (ratio of plasma to magnetic pressures) increasing above 0.05 (ref. 37 ) and |z_gsm|<5 Re . Only data from August 01 to October 08 (for 2002, 2003 and 2004), when |y_gsm|<10 Re , were used to exclude magnetopause boundary layer excursions. Additionally, event selection was made according to the particle energy flux in the lobe: we require that the energy band between 700 ev and 2 keV, and at least one order of magnitude for all energy bands, contain a particle energy flux greater than 8 × 10 4 keVs −1 cm −2 si −1 keV −1 . Based on these criteria, only events with magnetosheath or cusp-like [35] , [36] ions with energy around 1 keV were selected, and the upflowing ions with lower energy [29] , [34] from the ionosphere were excluded. The spatial distribution of all-of-the events is plotted in Fig. 1 . We find that the selected events are distributed at the high-latitude magnetosphere and around the mid-night sector. A total of 104 events was found, with 45 and 59 occurring in the southern and northern hemispheres, respectively. 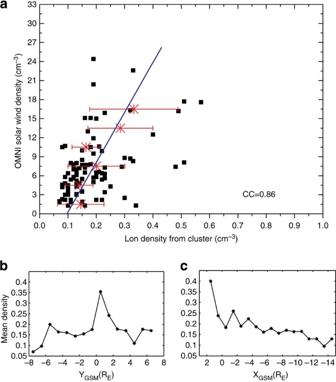Figure 3: Ion densities of the entry plasmas. (a) Ion densities for the events versus the corresponding solar wind density. Black markers indicate the events, whereas red stars are the average value for each 3-SW density bin with more than 3 points. (Two extreme events that exhibited densities of greater than 1 are not shown here.) The positive relationship between the average density and solar wind density strongly indicates that the entry plasmas are originated from the (compressed) solar wind. Mean ion density values along (b) they-direction and (c) thex-direction for each 1-Re-bin, respectively. The density was higher near the mid-night sector and, therefore, the contribution of K-H instability25,26and gradient drift processes27at low latitudes can be excluded. Figure 3a shows that the plasma density of these events is greater than 0.05 cm −3 , which is much higher than the lobe background level [29] , [34] . The bulk ion flow speeds are below 60 km s −1 (not shown). The ion temperature for most of the events is <20 MK, which is lower than that in the normal magnetotail plasma sheet (typically greater than 60 MK) but very close to that in the cusp or magnetosheath. Figure 3a also shows that higher solar wind densities correspond to the higher ion densities observed by Cluster. The above evidence further supports the point that these ions enter from the solar wind or from the magnetosheath. Furthermore, the Kp index, an indicator frequently used to weigh the disturbance levels of the geomagnetic field, has been found to be <3 during most of the events. Therefore, we call these regions with incoming solar wind plasmas ‘entry regions’ at the nightside high-latitude magnetosphere during geomagnetic (nearly) quiet periods. For more than half of the events (63), we could determine spatial regions when multi-point ion or electron density profiles were available onboard Cluster using the technique we mentioned above [35] , [36] . Figure 3: Ion densities of the entry plasmas. ( a ) Ion densities for the events versus the corresponding solar wind density. Black markers indicate the events, whereas red stars are the average value for each 3-SW density bin with more than 3 points. (Two extreme events that exhibited densities of greater than 1 are not shown here.) The positive relationship between the average density and solar wind density strongly indicates that the entry plasmas are originated from the (compressed) solar wind. Mean ion density values along ( b ) the y -direction and ( c ) the x -direction for each 1-Re-bin, respectively. The density was higher near the mid-night sector and, therefore, the contribution of K-H instability [25] , [26] and gradient drift processes [27] at low latitudes can be excluded. Full size image We now consider how these entry regions are formed. Firstly, we examined the IMF conditions for all the events. 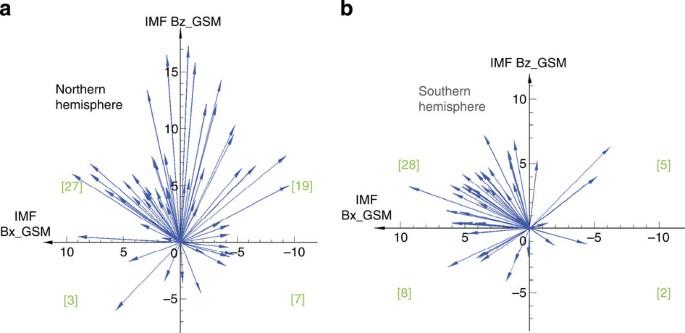Figure 4: IMF vectors for the events. (a) IMF vectors for the events that were observed in the northern hemisphere (59 events); (b) IMF vectors for the events that were observed in the southern hemisphere (45 events). Most events (84) occurred when the IMF was directed northerly, whereas only 20 events occurred when the IMF was southward, of which nine occurred during or within 10 min after the IMF turned from north to south, three occurred when the IMF turned within 1.5 h, and the rest occurred during time periods with an unstable IMF. The IMF Bx behaviour was very different for the events in the NH and SH, which can be well explained by the scenario illustrated inFig. 1. Figure 4 shows that most of the events occurred when the IMF had a northward orientation. This result is very remarkable because, while Cluster was traversing the whole lobe region in each pass, the durations of the northerly and southerly directed IMF were approximately equal; however, most events occurred just for those intervals where the IMF was northward. It is well known that when the IMF is northward, at high latitudes the K-H instability [25] , [26] , a process that is believed to dominate plasma transport at low latitudes, is unlikely to occur, because the instability is stabilized by the magnetic field along the flow direction. A northward IMF, however, provides a precondition for MR [10] , [30] , [38] , [39] between the antiparallel magnetic field lines of the solar wind and the magnetosphere at the high-latitude magnetopause. If MR occurs, then the magnetosphere could be opened there so that the process transports plasma into the lobe. Thus, one may infer that high-latitude reconnection at the magnetopause can account for these events. Figure 4: IMF vectors for the events. ( a ) IMF vectors for the events that were observed in the northern hemisphere (59 events); ( b ) IMF vectors for the events that were observed in the southern hemisphere (45 events). Most events (84) occurred when the IMF was directed northerly, whereas only 20 events occurred when the IMF was southward, of which nine occurred during or within 10 min after the IMF turned from north to south, three occurred when the IMF turned within 1.5 h, and the rest occurred during time periods with an unstable IMF. The IMF Bx behaviour was very different for the events in the NH and SH, which can be well explained by the scenario illustrated in Fig. 1 . Full size image Further evidence supporting this scenario can be derived from the different IMF orientations for the events in each hemisphere ( Fig. 4 ). For the events in the northern hemisphere, the number of events with a positive IMF Bx was nearly the same as that with a negative IMF Bx, whereas for the events in the southern hemisphere, more events occurred when the IMF Bx values were positive. A possible explanation is provided by Fig. 1 , which shows that during the season August to October the Earth’s magnetic dipole axis tilted towards the Sun for most of the time, so that the magnetic equator was typically inclined as indicated, resulting in lobe field lines in the northern hemisphere lying much closer to the draped IMF after it passes through the bow shock, as shown. A number of authors [39] , [40] have suggested that the dipole tilt, and not the IMF tilt (or IMF Bx), determines in which hemisphere high-latitude reconnection first occurs, because the IMF tilt angle effect will be weakened by the magnetic field draping at the magnetopause. Therefore, a sunward dipole tilt favours initial MR at the northern hemisphere irrespective of whether the IMF Bx values are positive or negative. We were thus able to identify events in the northern hemisphere under both positive and negative Bx conditions. As the draping effect is weaker in the southern hemisphere, however, MR will occur more readily there only when there is a sufficiently positive Bx, such that it would be more likely to find events in the southern hemisphere. For this reason, most events in the southern hemisphere were found under positive Bx conditions. Thus, this result may provide more evidence that these entry regions are produced by the high-latitude reconnection. Analysis of data from a different season (January to April of 2001–2003) supports the view that this kind of entry ions is found more likely under northward IMF. Although the number of events is small for a statistical study, we can still find some trends showing that, during the negative dipole tilt condition, the event number for positive and negative IMF Bx events in the southern hemisphere is balanced, which is consistent with our point above. It is known that other processes such as the K-H instability [25] , [26] or gradient drift processes [27] tend to occur near the flanks and this is likely to source entry plasma predominantly in the low-latitude flank regions. The mean plasma density, however, is higher near the local mid-night at high latitudes ( Fig. 3b ). This further confirms that the entry plasmas in our observations is unlikely to be sourced by those mechanisms operating at low latitudes (K-H instability at the high latitudes may still operate under some special conditions [41] ), and are more consistent with the near mid-night operation of the high-latitude reconnection. The entry region locations at the high latitude that are predicted by the simulations (the yellow or green regions of Fig. 2(6) of Li et al. [22] ) are very well consistent with our observations. Moreover, the density is higher at the near-Earth locations ( Fig. 3c ), wherein the lobe reconnection is thought to be more likely to occur. Such a density profile is consistent with Li et al. ’s [21] MHD simulation study ( Fig. 2b in their paper). Woch and Lundin [23] , [24] in their previous work advocate direct impulsive entry mechanism of magnetosheath plasma into the magnetosphere in the regions in the vicinity of the cusp. As Viking was at very low altitudes on the nightside, they claimed that there were no indications of entry ions occurring near the mid-night region. Therefore our work, which concentrates on the entry regions in the high latitude and high altitude part of the magnetosphere (mostly on the nightside), could be new developments of these previous works. The statistical result of IMF conditions by Woch and Lundin [24] differs significantly to ours, however: they found most events happened under horizontal IMF direction while most of ours are under vertical (northward) IMF. Woch and Lundin [23] , [24] proposed that solar wind plasma enters the magnetosphere locally and sporadically by crossing the magnetopause discontinuity in the absence of magnetic field merging (calling this ‘impulsive penetration’ [42] ). Comparing with Woch and Lundin’s statistical work [24] , in which they have found that some of the most prominent events are related to plasma irregularities in the solar wind, as the impulsive penetration mechanism [42] predicts, we did not find significant changes of solar wind properties from the OMNI data for most of our events, and only a few events ( ∼ 12 cases) were related to the IMF turning from north to south, which might be related to this mechanism. However, the solar wind may have had some local irregularities near the earth. Therefore, in this paper we cannot totally rule out the possibility of impulsive penetration mechanism for a few of the events, although it cannot explain the dominant northward IMF situation and the north–south hemisphere asymmetry of the events we found. As the most important point of this paper is on the new observations of solar wind entry regions, we are open to any mechanisms other than high latitude MR. And it could be studied in the future to what extent impulsive penetration (and other) processes contribute to our events. Finally, we note that the solar wind entry rate can be estimated using the total number of particles divided by the entry time for each event. The former can be calculated as ∼ ( V perp t ) 2 ·L·n , where V perp is the average perpendicular velocity of each event, t is the crossing time, L is the length of the regions (assuming ∼ 20 Re here) and n is the average density of the event. If these particles enter within 1 min (observed periodicity of pulsed reconnection at the high-latitude magnetopause [43] ), the entry rate can be estimated to be of the order of between 10 24 and 10 27 particles per second for different events. The upper value is comparable to estimations of entry rates during active times [7] , [44] , and also consistent with recent global MHD simulation results [22] of 10 26 –10 27 particles per second during northward IMF. If reconnection is continuous [45] instead of pulsed, the entry process will be continuous and then the entry rate can be even larger. Thus, this region could be the primary region for solar wind plasma entry from the magnetosheath to the magnetosphere during geomagnetically quiet times. The potential global relationship of the entry processes, for example, to the auroral regions and the magnetotail plasma sheet, are open questions and should be studied in future work. In fact a large body of simultaneous coverage of both high and low latitudes are available through the recent operation of many spacecraft distributed around the magnetosphere (for example, Time History of Events and Macroscale Interactions during Substorms (THEMIS), Double Star and Geotail/Wind) or with future missions, such as MMS. How to cite this article: Shi, Q. Q. et al. Solar wind entry into the high-latitude terrestrial magnetosphere during geomagnetically quiet times. Nat. Commun. 4:1466 doi: 10.1038/ncomms2476 (2013).